Smart responsive phosphorescent materials for data recording and security protection Smart luminescent materials that are responsive to external stimuli have received considerable interest. Here we report ionic iridium (III) complexes simultaneously exhibiting mechanochromic, vapochromic and electrochromic phosphorescence. These complexes share the same phosphorescent iridium (III) cation with a N-H moiety in the N^N ligand and contain different anions, including hexafluorophosphate, tetrafluoroborate, iodide, bromide and chloride. The anionic counterions cause a variation in the emission colours of the complexes from yellow to green by forming hydrogen bonds with the N-H proton. The electronic effect of the N-H moiety is sensitive towards mechanical grinding, solvent vapour and electric field, resulting in mechanochromic, vapochromic and electrochromic phosphorescence. On the basis of these findings, we construct a data-recording device and demonstrate data encryption and decryption via fluorescence lifetime imaging and time-gated luminescence imaging techniques. Our results suggest that rationally designed phosphorescent complexes may be promising candidates for advanced data recording and security protection. Data recording, storage and security technologies have been widely utilized in economic and military fields as well as in our daily life. Smart luminescent materials that are responsive to external stimuli have received considerable attention in the construction of optical data recording and storage devices [1] , [2] , [3] , [4] , [5] . These materials have been classified on the basis of the types of external stimuli that they are responsive to. Mechanochromic materials show changes in emission colour in the presence of mechanical stimuli (for example, shearing, grinding and rubbing) because of the interruption of intermolecular interactions (for example, π-π stacking and hydrogen bonds) [6] , [7] , [8] , [9] , [10] . Vapochromic luminescence has been observed in materials that are responsive to volatile organic compounds [11] , [12] . Electric field is an important external stimulus. Electrochromism occurs in π-conjugated polymers because of the reversible transition between two redox states [13] , [14] , [15] , [16] . However, materials showing electrochromic luminescence, which is distinct luminescence colour responses to an electric field, are scarce. We envision the potential commercial applications of electrochromic luminescent materials because they can be conveniently integrated into semiconductor-based electronic devices. In addition, it is conceivable that compounds simultaneously showing mechanochromic, vapochromic and electrochromic luminescence are of great use to the development of multifunctional materials. Phosphorescent transition–metal complexes, such as those of Ir(III) and Pt(II), have been extensively studied for various photonic and electronic applications because of their rich excited-state properties, including high luminescence quantum yields, long emission lifetimes, large Stokes shifts, high photostability and various luminescence colours [17] , [18] , [19] , [20] . These complexes have also been utilized as external stimuli-responsive materials because of their highly sensitive photophysical properties to the microenvironment [21] , [22] , [23] . In addition, the long-lived phosphorescence of these complexes renders them suitable for a time-resolved luminescence technique, which is incompatible with short-lived fluorescent dyes [24] , [25] . In view of these interesting phosphorescence properties, in particular their high sensitivity to external stimuli and long phosphorescence lifetime, we believe that transition–metal complexes have a great potential to serve as materials for optical data recording and security protection. In this study, we report a series of ionic Ir(III) complexes sharing the same phosphorescent Ir(III) cation with a N-H moiety in the N^N ligand and containing different counterions including PF 6 − , BF 4 − , I − , Br − and Cl − . The anionic counterions cause a variation in the emission colours of the complexes by forming hydrogen bonds with the N-H proton. Interestingly, the emission colours of these complexes are sensitive to mechanical, volatile organic compounds and electrical stimuli, all of which influence the electronic effect of the N-H moiety in the N^N ligand. On the basis of our findings, a quasi-solid data recording and storage device is fabricated to show the evident luminescence colour change from yellow to green at a low voltage. Owing to the advantageous long phosphorescence lifetime of the Ir(III) complexes, data encryption and decryption are demonstrated via the fluorescence lifetime imaging microscopy (FLIM) and time-gated luminescence imaging (TGLI) techniques. Synthesis and characterization of the Ir(III) complexes This study presents a universal approach that uses mechanochromic, vapochromic and electrochromic phosphorescence of Ir(III) complexes for data recording and security protection. Our designed complexes [ppy 2 IrNH] + A − (ppy=2-phenylpyridine, A − =PF 6 − ( 1 ), BF 4 − ( 2 ), I − ( 3 ), Br − ( 4 ) and Cl − ( 5 ), see Fig. 1a ) share the same phosphorescent Ir(III) cation with the N^N ligand, 2-(2-pyridyl)benzimidazole (NH), which contains a N-H moiety, the electronic effect of which is sensitive to external stimuli. Different anionic counterions (A − ) have been involved via anion exchange reactions. In addition, complexes [pq 2 IrNH] + A − (pq=2-phenylquinoline, A − =PF 6 − ( 6 ), I − ( 7 ), Br − ( 8 ) and Cl − ( 9 )) and [ppy 2 IrNEt] + A − (Et=ethyl, A − =PF 6 − ( 10 ) and Br − ( 11 )), in which ppy was replaced by a more conjugated pq ligand or the sensitivity of the N-H moiety was eliminated by an ethyl substitution, have also been synthesized for comparison study (see Fig. 1b ). 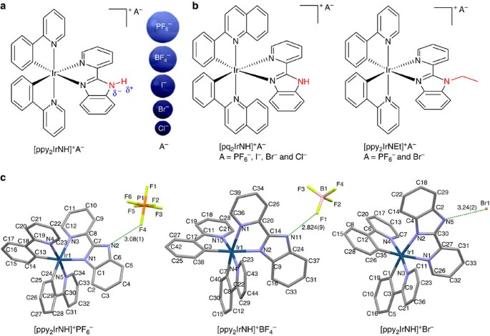Figure 1: Molecular structures and crystal structures. (a) Chemical structures of [ppy2IrNH]+A−. (b) Chemical structures of [pq2IrNH]+A−and [ppy2IrNEt]+A−. (c) Single-crystal structures of complexes [ppy2IrNH]+PF6−, [ppy2IrNH]+BF4−and [ppy2IrNH]+Br−, collected at 296 K. The complexes were characterized via FTIR, 1 H NMR, 13 C NMR, 19 F NMR, matrix-assisted laser desorption ionization time-of-flight mass spectrometry (MALDI-TOF MS), electrospray ionization mass spectrometry (ESI-MS), (see Supplementary Figs 1–11 ) X-ray crystal structure analysis (see Supplementary Data 1–4 and Supplementary Table 1 ), UV/Vis absorption spectrometry and steady-state fluorescence spectrometry. Figure 1: Molecular structures and crystal structures. ( a ) Chemical structures of [ppy 2 IrNH] + A − . ( b ) Chemical structures of [pq 2 IrNH] + A − and [ppy 2 IrNEt] + A − . ( c ) Single-crystal structures of complexes [ppy 2 IrNH] + PF 6 − , [ppy 2 IrNH] + BF 4 − and [ppy 2 IrNH] + Br − , collected at 296 K. Full size image The variation in the anionic counterions in [ppy 2 IrNH] + A − was confirmed using their X-ray single-crystal structures (see Fig. 1c ), 1 H NMR spectra (see Fig. 2a ) and FTIR spectra (see Supplementary Fig. 12 ). Single crystals of [ppy 2 IrNH] + PF 6 − , [ppy 2 IrNH] + BF 4 − and [ppy 2 IrNH] + Br − that are suitable for X-ray crystallography were obtained from addition of hexane to their CH 2 Cl 2 solution. 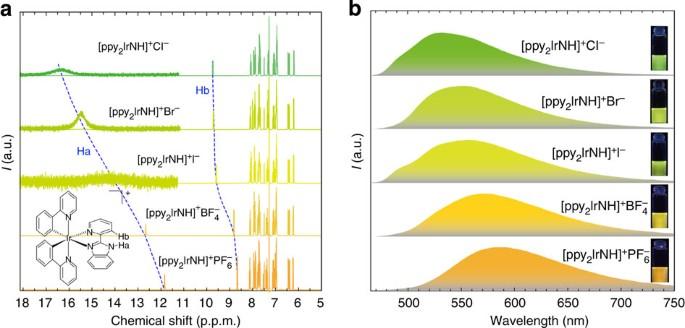Figure 2:1H NMR characterization and optical features. (a)1H NMR spectra of [ppy2IrNH]+A−in CDCl3. (b) Photoluminescence spectra of [ppy2IrNH]+A−in CH2Cl2at 296 K (10 μM,λex=365 nm). The insets show the photographs under a UV lamp. Supplementary Table 2 listed the selected bond lengths. Interestingly, multiple interactions such as hydrogen bonds and π-π stacking were observed in the single crystals (see Supplementary Figs 13–16 ). For example, in [ppy 2 IrNH] + PF 6 − , the N-H bond points towards one of the fluorine atoms of PF 6 − with a N2 … F4 distance of 3.08(1) Å, which indicates the presence of the N2-H … F4 hydrogen bond. In addition, π-π stacking occurs between benzimidazole rings of adjacent molecules with an interplanar separation of ~3.26 Å. In [ppy 2 IrNH] + BF 4 − and [ppy 2 IrNH] + Br − , a N11 … F1 distance of 2.824(9) Å and a N5 … Br1 distance of 3.24(2) Å were observed, respectively, which indicates the hydrogen-bonding interactions. Moreover, the chemical shifts of the N-H proton in 1 H NMR spectra indicated the formation of hydrogen bonds with the counterions in solution. The signal of this proton displayed a marked downfield shift when counterion changed from PF 6 − to Cl − , which is in agreement with the reported hydrogen bond-accepting capability of the anions in solutions (PF 6 − <BF 4 − <I − <Br − <Cl − ) [26] , [27] . Previous reports have also confirmed this observation that revealed the formation or strengthening of hydrogen bonds leads to a decrease in the electron density on the bonding hydrogen atom and an increase on the acceptor and donor heteroatoms [28] , [29] , [30] , thereby resulting in a downfield shift of the proton chemical shift [31] . Figure 2: 1 H NMR characterization and optical features. ( a ) 1 H NMR spectra of [ppy 2 IrNH] + A − in CDCl 3 . ( b ) Photoluminescence spectra of [ppy 2 IrNH] + A − in CH 2 Cl 2 at 296 K (10 μM, λ ex =365 nm). The insets show the photographs under a UV lamp. Full size image Counterion-dependent phosphorescence All the Ir(III) complexes exhibit intense and long-lived phosphorescence (see Supplementary Fig. 17 ) at room temperature upon photoexcitation. The photophysical data of the Ir(III) complexes have been summarized in Table 1 , and the photoluminescence spectra of the complexes (10 μM) in CH 2 Cl 2 at room temperature have been shown in Fig. 2b . The luminescence quantum yield of [ppy 2 IrNH] + I − was reduced compared with those of the other complexes, and this result has been tentatively attributed to the most significant heavy atom effect of iodine among halogen [32] . The variation in anionic counterions caused a negligible effect on the absorption spectra of the complexes (see Supplementary Fig. 18 ), but, interestingly, the emission wavelengths of the complexes varied from 588 to 532 nm. The counterion-induced emission colour change was probably caused by the N-H … X (X=halogen) hydrogen bond. As described in the 1 H NMR analysis, the strengthening of the N-H … X hydrogen bond reduces the electron cloud density of the bonding hydrogen, while the donor nitrogen atom gains electron cloud density, leading to the downfield shift of the proton signal of the N-H moiety as the counterions of [ppy 2 IrNH] + A − change from PF 6 − to Cl − (see Fig. 2a ). According to the theoretical calculation results, the highest occupied molecular orbital (HOMO) is located on the iridium centre and C^N ligand (ppy), and the lowest unoccupied molecular orbital (LUMO) is dominated by the N^N ligand (see Supplementary Fig. 19 ). Thus, increasing electron cloud density on the nitrogen atom of the N-H moiety will elevate the energy level of LUMO, but with tiny effect on HOMO. As such, [ppy 2 IrNH] + A − displayed a blue shift of the emission maximum when the counterion changed from PF 6 − to Cl − . In addition, electrochemical data (see Supplementary Fig. 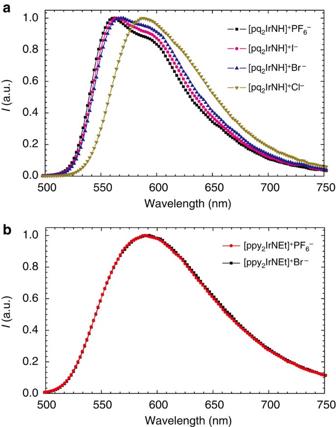Figure 3: Optical features of [pq2IrNH]+A−and [ppy2IrNEt]+A−. (a) Normalized photoluminescence spectra of [pq2IrNH]+A−in CH2Cl2at 296 K (10 μM,λex=365 nm). (b) Normalized photoluminescence spectra of [ppy2IrNEt]+A−in CH2Cl2at 296 K (10 μM,λex=365 nm). 20 and Supplementary Table 3 ) showed that the reversible Ir(IV/III) oxidation couples of all complexes occurred at ~0.87 V against ferrocene/ferricenium. The N^N ligand-based reduction waves were irreversible, and their potentials became more negative when the counterions of the complexes changed from PF 6 − through BF 4 − , I − , Br − to Cl − , which is in agreement with the change in emission wavelengths of the complexes. Table 1 Photophysical data for [ppy 2 IrNH] + A − in CH 2 Cl 2 (10 μM). Full size table To demonstrate the universality of the emission-tuning strategy, complexes [pq 2 IrNH] + A − have been designed. Their photoluminescence spectra in CH 2 Cl 2 solution (10 μM) are shown in Fig. 3a . Similar to the case of [ppy 2 IrNH] + A − , a counterion variation induced different emission colours of [pq 2 IrNH] + A − . However, the emission wavelength tuning range is smaller than that of the ppy analogues. The reasons are as follows: the luminescence of the ppy complexes originates from a triplet metal-to-ligand charge-transfer ( 3 MLCT) excited state with the LUMO dominated by the N^N ligand, while the emissive state of the pq complexes involves predominantly triplet intraligand ( 3 IL) character with both HOMO and LUMO located on the pq ligand. As a result, the formation of hydrogen bonds between counterions and the N^N ligand causes more significant effects on the emission properties of the ppy complexes. This explanation is further supported by the theoretical calculation results (see Supplementary Fig. 19 ), in which the emissive state of the ppy complexes is more closely related to the electronic property of N^N ligand than that of the pq complexes. Figure 3: Optical features of [pq 2 IrNH] + A − and [ppy 2 IrNEt] + A − . ( a ) Normalized photoluminescence spectra of [pq 2 IrNH] + A − in CH 2 Cl 2 at 296 K (10 μM, λ ex =365 nm). ( b ) Normalized photoluminescence spectra of [ppy 2 IrNEt] + A − in CH 2 Cl 2 at 296 K (10 μM, λ ex =365 nm). Full size image To demonstrate the function of the N-H moiety in the phosphorescence-tuning strategy, two control complexes [ppy 2 IrNEt] + A − have been synthesized (see Fig. 1b ). The replacement of hydrogen atom in the N-H moiety with an ethyl group eliminated the formation of hydrogen bonds, and the emission wavelengths of both complexes were almost the same (see Fig. 3b ). Mechanochromic and vapochromic phosphorescence [ppy 2 IrNH] + PF 6 − was selected to study the potential application of these Ir(III) complexes as mechanochromic materials. In the solid state, this complex exhibited green colour phosphorescence at 543 nm and has been named as [ppy 2 IrNH] + PF 6 − -G. Interestingly, grinding this complex on a quartz plate induced a red-shift of the emission maximum to 585 nm and yielded a yellow-emitting powder [ppy 2 IrNH] + PF 6 − -Y (see Fig. 4a ). Since similar phosphorescence colour change has not been observed when a pressure of 20 MPa is applied to an IR pellet press containing [ppy 2 IrNH] + PF 6 -G (see Supplementary Fig. 21 ), the mechanochromic behaviour probably results from the shearing force. Interestingly, exposing this powder to a solvent vapour of CH 2 Cl 2 , CHCl 3 or THF for several seconds will revert the emission colour to green because of vapour-induced recrystallization [33] . A rewritable data recording device has been constructed (see Fig. 4b ) based on the reversible mechanochromism and vapochromism of [ppy 2 IrNH] + PF 6 − . This complex was grinded and coated on a quartz plate as the ‘paper’, on which a word ‘IAM’ was written using a specially made ‘pen’ with CH 2 Cl 2 vapour as the ‘ink’. In contrast to the yellow-emitting background, the word ‘IAM’ showed intense green emission. This word can similarly be easily erased by grinding, and the writing and erasing processes can be repeated. 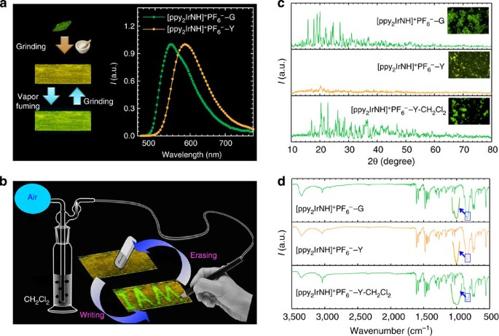Figure 4: Mechanochromic and vapochromic experiments. (a) Luminescence photographs and photoluminescence spectra of [ppy2IrNH]+PF6−before ([ppy2IrNH]+PF6−-G) and after ([ppy2IrNH]+PF6−-Y) grinding. (b) The constructed rewritable data recording device based on mechanochromic and vapochromic phosphorescence. (c) Power X-ray diffraction patterns of the corresponding samples. (d) FTIR spectra of the corresponding samples. Figure 4: Mechanochromic and vapochromic experiments. ( a ) Luminescence photographs and photoluminescence spectra of [ppy 2 IrNH] + PF 6 − before ([ppy 2 IrNH] + PF 6 − -G) and after ([ppy 2 IrNH] + PF 6 − -Y) grinding. ( b ) The constructed rewritable data recording device based on mechanochromic and vapochromic phosphorescence. ( c ) Power X-ray diffraction patterns of the corresponding samples. ( d ) FTIR spectra of the corresponding samples. Full size image The complete consistency of the characterization data ( 1 H NMR and MALDI-TOF MS) of [ppy 2 IrNH] + PF 6 − -G and [ppy 2 IrNH] + PF 6 − -Y (see Supplementary Figs 1, 22 and 23 ) indicated that no change occurred in the molecular structure of the complex during grinding. The difference in the phosphorescence colours has been attributed to the change in the molecular packing mode and intermolecular interactions. To understand the possible origin of this behaviour, the powder X-ray diffraction (PXRD) of the samples was studied. The PXRD patterns and the fluorescence microscopy images of the corresponding samples have been shown in Fig. 4c . PXRD patterns of [ppy 2 IrNH] + PF 6 − -G showed intense and sharp reflection peaks, which indicated that the aggregate was well ordered. By contrast, [ppy 2 IrNH] + PF 6 − -Y showed very weak and broad diffraction signals, suggestive of an amorphous or partially amorphous state. After fuming the [ppy 2 IrNH] + PF 6 − -Y with CH 2 Cl 2 vapour, the diffraction peaks of the complex (named as [ppy 2 IrNH] + PF 6 − -Y-CH 2 Cl 2 ) reappeared (see Fig. 4c ), which suggested that the crystalline state was recovered through molecular repacking. Considering the significant function of hydrogen bonds in the phosphorescence colour tuning of [ppy 2 IrNH] + A − in solution, the green emission of well-ordered [ppy 2 IrNH] + PF 6 − -G has been tentatively attributed to the hydrogen bond between PF 6 − and the N^N ligand, which was observed in the single-crystal structure (see Fig. 1c and Supplementary Fig. 13 ). As a weak molecular interaction, hydrogen bonding is easily broken and rebuilt at specific external stimuli [34] . Hence, the mechanochromism and vapochromism of [ppy 2 IrNH] + PF 6 − were probably caused by the breaking and restoring of hydrogen bonds when the complex was subjected to mechanical grinding and exposed to CH 2 Cl 2 vapour. To further investigate the effect of external stimuli on hydrogen bonds, FTIR measurements have been performed, which has been widely used to study hydrogen bonds in supramolecular self-assembly [35] . The FTIR spectra of [ppy 2 IrNH] + PF 6 − -G, [ppy 2 IrNH] + PF 6 − -Y and [ppy 2 IrNH] + PF 6 − -Y-CH 2 Cl 2 have been shown in Fig. 4d . Generally, PF 6 − displays a monomodal F-P stretching peak around 841 cm −1 in the FTIR spectrum. However, the F-P stretching peak was split into two bands at 854 and 838 cm −1 for [ppy 2 IrNH] + PF 6 − -G and [ppy 2 IrNH] + PF 6 − -Y-CH 2 Cl 2 , and this result has been attributed to the inequivalence of the six F-P bonds caused by the N-H … F hydrogen bond. Only one F-P stretching peak at 841 cm −1 was observed for [ppy 2 IrNH] + PF 6 -Y because the hydrogen bond vanished. The PXRD data, single-crystal structures and FTIR spectra showed that the observed mechanochromic and vapochromic phosphorescence originated from variations in the molecular packing mode and hydrogen bonds between the counterion and the ligand. Electrochromic phosphorescence The response of [ppy 2 IrNH] + PF 6 − towards an electrical stimulus has been analysed via electrochromic phosphorescence experiments, because the phosphorescence properties of [ppy 2 IrNH] + A − are strongly related to the electronic effect of the N-H moiety. As illustrated in Fig. 5a , two tin electrodes were immersed in a CH 3 CN solution of [ppy 2 IrNH] + PF 6 − (200 μM) with a distance of 20 mm between each other. Before applying a voltage, the solution exhibited yellow emission (see Fig. 5a ). At voltages higher than 10 V, the emission colour of the solution near the anode remained yellow all throughout. However, green emission was observed near the cathode within several seconds (see Fig. 5a ) and gradually extended to the middle of the two electrodes, which revealed a clear boundary (see Fig. 5a and Supplementary Movie 1 ). This process took several minutes to reach equilibrium depending on the magnitude of the applied voltage. The green emission returned back to yellow upon stirring and reappeared when the stirring was stopped. This phenomenon can be observed repeatedly. Interestingly, when the distribution of the applied electric field was modulated by an additional tin plate placed between the two electrodes, both the separated cells exhibited the similar phenomenon (see Fig. 5a and Supplementary Fig. 24 ). The interesting electrochromic phosphorescence can be applied to patterning by controlling the distribution of the electric field. 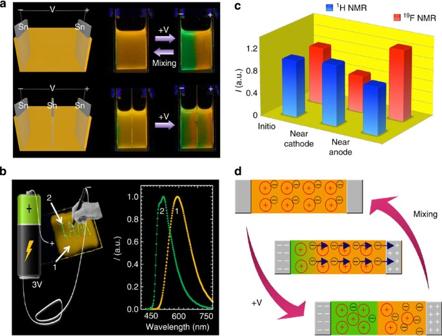Figure 5: Electrochromic phosphorescence experiments. (a) The setup used for electrochromic phosphorescence experiments and the photographs of electrochromic phosphorescence of [ppy2IrNH]+PF6−(200 μM) in CH3CN. (b) Quasi-solid film under a UV lamp. Inset: the emission spectra of [ppy2IrNH]+PF6−(λex=365 nm) before (1) and after (2) applying a voltage in quasi-solid device. (c) Concentration variation of [ppy2IrNH]+and PF6−based on the1H NMR and19F NMR spectra. (d) Schematic illustration of the migration and distribution of ions under an electric field. Figure 5: Electrochromic phosphorescence experiments. ( a ) The setup used for electrochromic phosphorescence experiments and the photographs of electrochromic phosphorescence of [ppy 2 IrNH] + PF 6 − (200 μM) in CH 3 CN. ( b ) Quasi-solid film under a UV lamp. Inset: the emission spectra of [ppy 2 IrNH] + PF 6 − ( λ ex =365 nm) before (1) and after (2) applying a voltage in quasi-solid device. ( c ) Concentration variation of [ppy 2 IrNH] + and PF 6 − based on the 1 H NMR and 19 F NMR spectra. ( d ) Schematic illustration of the migration and distribution of ions under an electric field. Full size image The electrochromic phosphorescence did not originate from redox reactions because no change in emission colour was observed in the cyclic voltammetry experiment of [ppy 2 IrNH] + PF 6 − (see Supplementary Movie 2 ). The Ir(III) complexes near the two electrodes have been characterized to understand the origin of the electrochromic phosphorescence. The 1 H NMR and MS results showed that the structures of the complexes remained unchanged at our experimental conditions (see Supplementary Figs 25 and 26 ). On applying a voltage of 15 V for 3 min, the concentration of the Ir(III) complex cation increased by 10% near the cathode and decreased by 9% near the anode based on the integrals in the 1 H NMR spectra (see Fig. 5c ). The 19 F NMR spectra revealed that the concentration change of PF 6 − was much more significant; the concentration decreased markedly by 35% near the cathode and increased by 26% near the anode (see Fig. 5c,d and Supplementary Fig. 27 ). As a result, the non-homogeneous distribution of the ions led to the formation of a strong internal electric field near the cathode [36] . Therefore, the phosphorescence colour change of the solution near the cathode is probably caused by the polarization of the N-H bond under the internal electric field. Similar observation was absent in the control experiments, where the ethyl-substituted control complex [ppy 2 IrNEt] + PF 6 − was used (see Supplementary Fig. 28 ), thereby highlighting the significant function of the N-H moiety. A quasi-solid film has been fabricated by mixing [ppy 2 IrNH] + PF 6 − with ionic liquid BMIM + PF 6 − and silica nanoparticles to demonstrate the potential application of the interesting electrochromic phosphorescence for data recording and storage. The ionic liquid was employed because of its high ionic conductivity, thermal stability, negligible vapour pressure and wide electrochemical window [37] , [38] . The silica nanoparticles functioned as gelators to solidify the ionic liquid-based matrix through the supramolecular interaction (see Supplementary Fig. 29 ), with negligible influence on the migration of ions owing to the presence of the open channels [39] . Moreover, neither the BMIM + PF 6 − nor silica nanoparticles affected the phosphorescence properties of [ppy 2 IrNH] + PF 6 − (see Supplementary Figs 30 and 31 ). In this experiment, the fabricated film was sandwiched between an indium-tin oxide (ITO) anode and a movable Pt needle cathode. The handheld needle electrode functioned as a ‘pen’ to ‘write’ the word ‘IAM’ on the quasi-solid film. The film showed evident emission colour change from yellow to green at the point of ‘writing’ under a voltage as low as 3 V (see Fig. 5b ). Compared with the case in solution, the quasi-solid device required a much lower working voltage due to the rapid formation of the non-homogeneous distribution of ions because the BMIM + PF 6 − ionic liquid provided extra PF 6 − anions. Data encryption and decryption In addition to data recording, information encryption and decryption are important and have received considerable interest among scholars. A new strategy has been designed to achieve this objective. In the encryption process, a fluorescent dye is used to provide short-lifetime interference fluorescence (SLIF) into which the phosphorescence from [ppy 2 IrNH] + PF 6 − is completely embedded (see Fig. 6a ). For decryption, FLIM is used to highlight long-lived phosphorescence from [ppy 2 IrNH] + PF 6 − , or TGLI is employed to filter off short-lived fluorescence from the fluorescent dye. Our idea has been successfully supported and was confirmed by experimental results. The boron-dipyrromethene (BODIPY) dye (see Supplementary Fig. 32 ) has been selected to provide SLIF because of its intense fluorescence ( Φ =0.65), short lifetime ( τ =5 ns) and no efficient electronic communication with [ppy 2 IrNH] + PF 6 − (see Supplementary Figs 33 and 34 ). The steady-state emission spectrum of a mixture of the BODIPY dye (100 μM) and [ppy 2 IrNH] + PF 6 − (10 μM) in BMIM + PF 6 − is dominated by the intense emission band of the BODIPY dye, and the emission from [ppy 2 IrNH] + PF 6 − is barely observed (see Supplementary Fig. 33d ). After a delay of 100 ns, the emission of [ppy 2 IrNH] + PF 6 − appeared (see Supplementary Fig. 33d ). On the basis of these observations, the BODIPY dye was added to the quasi-solid film containing [ppy 2 IrNH] + PF 6 − , forming the ‘security paper’, which has been placed on a probe station equipped with a needle electrode (see Fig. 6a and Supplementary Fig. 35 ). After writing a character ‘A’ by using the needle electrode ‘pen’ on the ‘security paper’, the recorded data were encrypted by the SLIF and could not be observed using a common fluorescent microscopy (see Fig. 6b ). To decrypt the data, FLIM was used to differentiate the character ‘A’ from the background by using the emission lifetime instead of the intensity as the reading signal because the lifetime of [ppy 2 IrNH] + PF 6 − (189 ns) was much longer than that of the BODIPY dye (5 ns) (see Fig. 6b ). Alternatively, as shown in the time-gated luminescence images (see Fig. 6c ), after exerting a delay time of 12 ns, the data ‘A’ became readable. With an increase in the delay time, the signal-to-noise ratio was further enhanced and the recorded ‘A’ became progressively clearer. The results demonstrate the advantages of phosphorescence signals in data recording and security protection, which can be applied to the production of secret media, such as identity documents and banknotes. 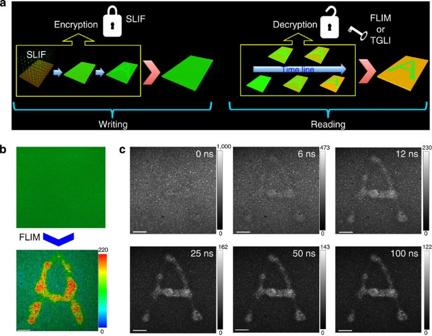Figure 6: Data encryption and decryption experiments. (a) Schematic diagram of information encryption and decryption. (b) Photoluminescence and fluorescence lifetime microscopy images (scale bar: average emission lifetime (ns): scale bar (length scale), 500 μm). (c) Time-gated luminescence images with different delay time (scale bar: emission intensity (counts): scale bar (length scale) 500 μm). Figure 6: Data encryption and decryption experiments. ( a ) Schematic diagram of information encryption and decryption. ( b ) Photoluminescence and fluorescence lifetime microscopy images (scale bar: average emission lifetime (ns): scale bar (length scale), 500 μm). ( c ) Time-gated luminescence images with different delay time (scale bar: emission intensity (counts): scale bar (length scale) 500 μm). Full size image In this work, we have designed and synthesized a series of ionic Ir(III) complexes containing a N-H moiety in their N^N ligand. Their different counterions cause a variation in the emission colours from yellow to green by forming hydrogen bonds with the N-H proton. Interestingly, these complexes respond to multiple types of external stimuli including mechanical force, solvent vapour and electric field, resulting in mechanochromic, vapochromic and electrochromic luminescence. On the basis of the mechanochromic and vapochromic phosphorescence of the complexes, a rewritable data recording device has been constructed by using CH 2 Cl 2 vapour as the ‘ink’ and mechanical grinding as the ‘eraser’ for data ‘recording’ and ‘erasing’, respectively. A quasi-solid data-recording device has been constructed using the needle electrode as an electric ‘pen’ based on the unexpected electrochromic phosphorescence of the complexes, and data encryption in the presence of the background fluorescence interference has been demonstrated. Meaningfully, data decryption has been achieved by utilizing FLIM and TGLI techniques, in which the long-lived phosphorescence of Ir(III) complexes plays an important role. We anticipate that phosphorescent transition–metal complexes will be promising candidates for applications in optical data recording and security protection technology by combining advanced optical imaging techniques. Materials Unless otherwise stated, all starting materials and reagents were purchased from commercial suppliers and were used without further purification. Silica particles (Aesoil 200, 12 nm) were purchased from Degussa Company (Evonik Industries AG, Rellinghauser Straβe 1-11, 45128 Essen, Germany). The fluorescent BODIPY dye was synthesized by our group, and its chemical structure was shown in Supplementary Fig. 32 . CH 2 Cl 2 , CH 3 CN and CDCl 3 were dried under reflux over CaH 2 for several hours at 70–75 °C, distilled at these conditions and used freshly. Synthesis and characterization of the complexes A mixture of 2-(2-pyridyl)benzimidazole (39 mg, 0.2 mmol) and [Ir(ppy) 2 ( μ -Cl)] 2 (107 mg, 0.1 mmol) in CH 2 Cl 2 /MeOH (24 ml, 3:1, v/v) was heated under reflux in a nitrogen atmosphere with stirring for 4 h. After the clear yellow solution was cooled down to room temperature, KPF 6 (368 mg, 2 mmol) was added. The suspension was stirred for 2 h and filtered to remove insoluble salts. The filtrate was evaporated to dryness under reduced pressure, and the crude product was purified via column chromatography (CH 2 Cl 2 /acetone) over silica gel to give [ppy 2 IrNH] + PF 6 − as yellow crystals. [ppy 2 IrNH] + BF 4 − , [ppy 2 IrNH] + I − , [ppy 2 IrNH] + Br − and [ppy 2 IrNH] + Cl − were obtained through ion exchange reactions of [ppy 2 IrNH] + PF 6 − with NaBF 4 , KI, NaBr and NaCl, respectively, in CH 2 Cl 2 /MeOH (3:1, v/v) with stirring at room temperature for 2 h, followed by column chromatography (CH 2 Cl 2 /acetone) over silica gel and recrystallization from CH 2 Cl 2 /hexane. [ppy 2 IrNH] + PF 6 − : (Yield, 50%). 1 H NMR (400 MHz, CDCl 3 ): δ =11.81 (s, 1H, NH), 8.65 (d, J =8.0 Hz, 1H, Ar), 8.10 (t, J =7.8 Hz, 1H, Ar), 7.96–7.82 (m, 4H, Ar), 7.80–7.62 (m, 5H, Ar), 7.48 (d, J =5.6 Hz, 1H, Ar), 7.42–7.32 (m, 2H, Ar), 7.13–7.03 (m, 2H, Ar), 7.03–6.91 (m, 5H, Ar), 6.45–6.40 (m, 1H, Ar), 6.40–6.35 (m, 1H, Ar), 6.22 (d, J =8.4 Hz, 1H, Ar). 13 C NMR (100 MHz, CDCl 3 ): δ =168.23, 167.92, 152.02, 150.75, 150.73, 149.51, 148.33, 147.66, 146.48, 144.05, 143.92, 140.09, 139.65, 137.85, 137.71, 134.35, 132.37, 131.76, 130.81, 130.17, 127.70, 126.48, 125.25, 124.78, 124.52, 124.36, 123.30, 122.99, 122.59, 122.50, 119.37, 119.34, 117.34, 114.56. MS (ESI) ( m/z ): calculated for C 34 H 25 IrN 5 696.17, found 696.25 [M + ]. [ppy 2 IrNH] + BF 4 − : (Yield, 56%). 1 H NMR (400 MHz, CDCl 3 ): δ =12.60 (s, 1H, NH), 8.78 (d, J =8.1 Hz, 1H, Ar), 8.12–8.04 (m, 1H, Ar), 7.94–7.82 (m, 4H, Ar), 7.78–7.63 (m, 5H, Ar), 7.47 (d, J =5.8 Hz, 1H, Ar), 7.41–7.29 (m, 2H, Ar), 7.12–7.02 (m, 2H, Ar), 7.02–6.90 (m, 5H, Ar), 6.46–6.40 (m, 1H, Ar), 6.40–6.34 (m, 1H, Ar), 6.22 (d, J =8.3 Hz, 1H, Ar). 13 C NMR (100 MHz, CDCl 3 ): δ =168.25, 167.94, 152.28, 150.95, 150.58, 149.54, 148.34, 147.93, 146.63, 144.06, 143.95, 140.13, 139.65, 137.79, 137.64, 134.63, 132.38, 131.78, 130.78, 130.14, 127.55, 126.24, 125.07, 124.76, 124.72, 124.50, 123.25, 122.93, 122.54, 122.44, 119.33, 119.31, 117.23, 114.71. MS (ESI) ( m/z ): calculated for C 34 H 25 IrN 5 696.17, found 696.25 [M + ]. [ppy 2 IrNH] + I − : (Yield, 58%). 1 H NMR (400 MHz, CDCl 3 ): δ =16.00–12.40 (broad, 1H, NH), 9.55 (d, J =8.0 Hz, 1H, Ar), 8.10–8.01 (m, 2H, Ar), 7.94–7.82 (m, 3H, Ar), 7.77–7.62 (m, 5H, Ar), 7.50–7.45 (m, 1H, Ar), 7.38–7.28 (m, 2H, Ar), 7.12–7.01 (m, 2H, Ar), 7.01–6.89 (m, 5H, Ar), 6.46–6.41 (m, 1H, Ar), 6.40–6.35 (m, 1H, Ar), 6.20 (d, J =8.3 Hz, 1H, Ar). 13 C NMR (100 MHz, CDCl 3 ): δ =168.28, 167.98, 152.92, 151.37, 150.36, 149.56, 148.54, 148.35, 146.90, 144.07, 144.00, 140.19, 139.29, 137.71, 137.53, 135.15, 132.39, 131.82, 130.73, 130.08, 127.23, 126.18, 125.63, 124.72, 124.69, 124.46, 123.18, 122.83, 122.44, 122.35, 119.28, 119.27, 117.10, 114.74. MS (ESI) ( m/z ): calculated for C 34 H 25 IrN 5 696.17, found 696.33 [M + ]. [ppy 2 IrNH] + Br − : (Yield, 57%). 1 H NMR (400 MHz, CDCl 3 ): δ =16.30–14.50 (broad, 1H, NH), 9.66 (d, J =8.0 Hz, 1H, Ar), 8.07 (t, J =8.4 Hz, 1H, Ar), 7.97 (d, J =8.3 Hz, 1H, Ar), 7.92–7.82 (m, 3H, Ar), 7.77–7.62 (m, 5H, Ar), 7.47 (d, J =5.6 Hz, 1H, Ar), 7.36–7.27 (m, 2H, Ar), 7.12–7.01 (m, 2H, Ar), 6.99–6.89 (m, 5H, Ar), 6.46–6.41 (m, 1H, Ar), 6.41–6.35 (m, 1H, Ar), 6.19 (d, J =8.3 Hz, 1H, Ar). 13 C NMR (100 MHz, CDCl 3 ): δ =168.28, 167.98, 152.76, 151.41, 150.25, 149.54, 148.54, 148.34, 146.96, 144.08, 144.01, 140.05, 139.43, 137.69, 137.52, 134.92, 132.40, 131.82, 130.72, 130.07, 127.20, 126.39, 125.61, 124.71, 124.66, 124.45, 123.15, 122.79, 122.42, 122.33, 119.28, 119.26, 117.08, 114.73. MS (ESI) ( m/z ): calculated for C 34 H 25 IrN 5 696.17, found 696.33 [M + ]. [ppy 2 IrNH] + Cl − : (Yield, 53%). 1 H NMR (400 MHz, CDCl 3 ): δ =17.34–15.23 (broad, 1H, NH), 9.69 (d, J =8.0 Hz, 1H, Ar), 8.09–8.02 (m, 1H, Ar), 7.97–7.78 (m, 4H, Ar), 7.77–7.60 (m, 5H, Ar), 7.52–7.44 (m, 1H, Ar), 7.34–7.26 (m, 2H, Ar), 7.11–7.00 (m, 2H, Ar), 6.99–6.86 (m, 5H, Ar), 6.45–6.41 (m, 1H, Ar), 6.41–6.35 (m, 1H, Ar), 6.19 (d, J =8.4 Hz, 1H, Ar). 13 C NMR (100 MHz, CDCl 3 ): δ =168.30, 168.00, 153.01, 151.63, 150.14, 149.55, 148.83, 148.35, 147.13, 144.09, 144.04, 140.18, 139.43, 137.64, 137.46, 135.34, 132.41, 131.84, 130.69, 130.03, 127.05, 126.34, 125.37, 124.69, 124.48, 124.43, 123.10, 122.74, 122.37, 122.27, 119.25, 119.23, 117.01, 114.88. MS (ESI) ( m/z ): calculated for C 34 H 25 IrN 5 696.17, found 696.33 [M + ]. Theoretical calculations The calculation was performed using the Gaussian 09 suite of programs [40] . The optimizations of the complex structures were performed by using B3LYP DFT. The LANL2DZ basis set was used to treat the iridium atom, whereas the 6–31 G* basis set was used to treat all other atoms. The contours of the HOMO and LUMO were plotted. Crystal and powder sample preparation Typical preparation procedures are as follows. The single crystal of the complexes was grown from their dichloromethane solution mixed with hexane. Hexane (20 ml) was poured into the solution of [ppy 2 IrNH] + PF 6 − (30 mg) in CH 2 Cl 2 (20 ml). This mixture was allowed to settle for a few minutes. The precipitate was collected as the green emission powder [ppy 2 IrNH] + PF 6 − -G. Measurements NMR spectra were recorded on a Bruker Ultra Shield Plus 400 MHz NMR instrument ( 1 H: 400 MHz, 19 F: 377 MHz). Mass spectra were obtained on a LCQ Fleet ESI mass spectrometer or a Bruker autoflex MALDI-TOF/TOF mass spectrometer. Photoluminescence spectra were recorded on an Edinburgh FL920 spectrofluorometer system. The absolute quantum yields of the complexes were determined through an absolute method by employing an integrating sphere. Time-resolved fluorescence lifetime measurements were carried out by using time-correlated single-photon counting lifetime spectroscopy system Edinburgh FL920 with a semiconductor laser as the excitation source ( λ ex =379 nm). The quality of the fit has been judged by goodness-of-fit parameters such as χ 2 -test (<1.2). FTIR spectra were recorded on a Shimadzu IRPrestige-21 spectrometer. Single-crystal X-ray analysis was performed on a Bruker Smart Apex CCD diffractometer with graphite monochromated Mo-Kα radiation ( λ =0.71073) using the ω -2 θ scan mode. The structures were solved by direction methods and refined by full-matrix least-squares against F 2 for all data using SHELX-97 (SMART, SAINT, SADABS and SHELXTL, Bruker AXS Inc., Madison, 2000). All calculations and molecular graphics were carried out on a computer using the SHELX-2000 program package and Mercury 3.0. The powder diffraction data were recorded at room temperature on a Rigaku Dmax 2000 with Cu K α radiation and a D/teX Ultra detector covering 10–80 ° (2 θ ). The diffraction data were collected at 20 °C. Unless otherwise stated, all the mechanochromic, vapochromic and electrochromic phosphorescence experiments were carried out at room temperature. FLIM and TGLI The FLIM imaging setup was integrated with an Olympus IX81 laser scanning confocal microscopy. The fluorescence signal was detected using the confocal microscopy, and correlative calculation of the data was performed by professional software, which was provided by PicoQuant company. A 405-nm picosecond-pulsed diode laser (<1 μW) with 2.5 MHz repetition rate was used for excitation. The time-resolved emission signals were obtained via a TCSPC technique. Typically, the device with the written ‘A’ was put on the platform, and a 2 mm × 2 mm sample area consisting of 200 × pixels was scanned with an acquisition rate of 2 ms per pixel. TGLI were obtained by collecting fluorescence signals with different delay times based on the obtained FLIM images. Accession codes: The X-ray crystallographic coordinates for [ppy 2 IrNH] + PF 6 − (296 K), [ppy 2 IrNH] + PF 6 − (120 K), [ppy 2 IrNH] + BF 4 − (296 K) and [ppy 2 IrNH] + Br − (296 K) have been deposited at the Cambridge Crystallographic Data Centre (CCDC), under deposition number CCDC 958057, 981977, 958058 and 958059. These data can be obtained free of charge from The Cambridge Crystallographic Data Centre via www.ccdc.cam.ac.uk/data_request/cif . How to cite this article: Sun, H. et al. Smart responsive phosphorescent materials for data recording and security protection. Nat. Commun. 5:3601 doi: 10.1038/ncomms4601 (2014).